The benzaldehyde oxidation paradox explained by the interception of peroxy radical by benzyl alcohol Benzaldehyde readily undergoes autoxidation to form benzoic acid on exposure to air at room temperature. Yet it can be formed in high yield from, for example, benzyl alcohol by oxidation using a variety of procedures and catalysts. Here we report the evidence to resolve this apparent paradox. It is confirmed that benzyl alcohol (and a number of other alcohols), even at low concentrations in benzaldehyde, inhibits the autoxidation. Furthermore we report on the structural features required for inhibition. Electron paramagnetic resonance spin trapping experiments demonstrate that benzyl alcohol intercepts, by hydrogen atom transfer, the benzoylperoxy radicals that play a key role in benzaldehyde autoxidation. A similar inhibition effect has also been observed for the aliphatic octanal/1-octanol system. Selective oxidation is important in both academic research and in industry [1] . One of the biggest challenges in such oxidations is to prevent over-oxidation so as to stop the reaction at an intermediate stage. Thus, a goal of many investigations has been to increase the selectivity of the intermediate product(s), even at the expense of activity [2] , [3] , [4] . One well-studied group of systems that demonstrate this selective oxidation is the aerobic oxidation of primary alcohols to afford aldehydes, because aldehydes are important intermediates that find application in the synthesis of many pharmaceuticals, agrochemicals and perfumes [3] , [5] , [6] , [7] , [8] . Benzyl alcohol is one of the most widely studied substrates [6] , [9] , [10] . In the literature, many researchers have reported the aerobic oxidation of benzyl alcohol to benzaldehyde, using a variety of catalytic systems, including supported metal catalysts, with yields up to ~99% [9] , [10] , [11] , [12] , [13] , [14] , implying that further oxidation to give benzoic acid does not take place. For example, we recently reported the solvent-less, aerobic oxidation of benzyl alcohol to benzaldehyde using supported gold or gold–palladium nanoparticles as catalysts with a selectivity of 99% to benzaldehyde [6] , [15] , [16] , [17] , [18] . These nanoparticle-based catalysts have also been reported for the selective aerobic oxidation of many other alcohols including aliphatic alcohols like 1-octanol with a very high selectivity to octanal [6] , [19] . It has long been known that benzaldehyde spontaneously undergoes autoxidation to yield benzoic acid simply upon exposure to air at ambient temperature (~293 K) [2] . A common laboratory observation is the appearance of crystalline benzoic acid in bottles of benzaldehyde stored over a period of time. The presence of catalysts, such as transition-metal ions, or free radical initiators, such as benzoyl peroxide or azo-bis-isobutyronitrile, increases the rate of this oxidation [20] , [21] . Photochemical excitation also facilitates this transformation and the consensus is that this reaction is a radical chain process [22] , [23] , [24] . It is therefore logical to ask how benzyl alcohol can be partially oxidized to give benzaldehyde in very high yield even in the presence of oxidation catalysts that are active in promoting conversion of benzaldehyde into benzoic acid, in some cases at temperatures as high as 433 K in the presence of 10 bar O 2 pressure. The question has been posed previously and it has long been recognized that benzyl alcohol is one of a diverse group of organic molecules that can act as an inhibitor of benzaldehyde oxidation [25] . Investigations on the reactivity and stability of benzaldehyde, under oxidation conditions date back to the late 1920s; McNesby and Heller gave a comprehensive critical review of the early work in 1954 (ref. 26 ). A recent literature search on this question yielded very little evidence concerning the detailed mechanism of the inhibition. Authors have suggested a variety of explanations for the high selectivity to benzaldehyde when benzyl alcohol is oxidized, including: (a) preferential bonding of benzyl alcohol over benzaldehyde to the catalytic sites [27] , (b) solvent molecules (e.g. acetic acid) forming hydrogen bonds with intermediate peroxy radicals, reducing their reactivity and hence preventing further oxidation [25] and (c) component(s) of the catalyst selectively inhibiting the oxidation of aldehyde [28] . All these proposals have been made with less than adequate experimental proof while most are speculative in nature. This situation prompted us to approach the problem from a different perspective. Herein we investigate this interesting phenomenon by employing electron paramagnetic resonance (EPR) spectroscopy combined with the spin trapping methodology and demonstrate the role of free radicals in the autoxidation of benzaldehyde. We found that the presence of a very small amount of benzyl alcohol and other alcohols, with at least one C–H group active for hydrogen atom transfer, inhibits the oxidation of benzaldehyde to benzoic acid even under extreme conditions of high temperature and high O 2 pressure. In addition, we show the generality of this effect and the structural requirements of the molecules capable of suppressing over-oxidation of the aldehyde. Benzaldehyde oxidation The oxidation of pure benzaldehyde was conducted under conditions analogous to those employed in our previous studies of the aerobic benzyl alcohol oxidation [17] , [29] . Benzaldehyde was oxidized under solvent-less conditions without a catalyst at 353 K in a glass reactor under 1 atm pressure of O 2 . This resulted in the formation of a slurry containing crystalline material after ~4 min. Analysis of this slurry (GC on a solution in acetone) showed it to be a mixture of benzoic acid (15%) and unchanged benzaldehyde (85%). Recent reports [20] , [21] , that supported Au nanoparticles catalyse the oxidation of benzaldehyde by enhancing the formation of the intermediate acyl radicals, rule out the possibility that the supported gold–palladium catalyst used in our earlier work on benzyl alcohol oxidation is responsible for the inhibition of benzaldehyde oxidation. The only other component, which could prevent the further oxidation of benzaldehyde, is the remaining benzyl alcohol. A simple visual examination of benzaldehyde and benzyl alcohol mixtures exposed to air at room temperature for 90 min showed that benzyl alcohol quantities as low as 2% were sufficient to inhibit the appearance of benzoic acid crystals. GC analyses of reaction mixtures during the initial stages of oxidation are shown in Fig. 1 ; the analysis revealed that no other products were formed. These simple studies confirm Partenheimer’s observations that in benzyl alcohol oxidation catalysed by Co (III), benzoic acid production only begins to accelerate when the benzyl alcohol level in the reaction mixture falls below ~10% [25] . That a very small amount of benzyl alcohol, present in benzaldehyde, is evidently involved in preventing the oxidation of benzaldehyde to benzoic acid forms the premise for the more detailed studies presented below. 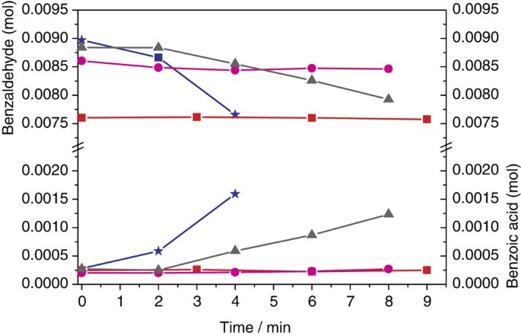Figure 1: Effect of benzyl alcohol on the aerobic oxidation of benzaldehyde. Reaction conditions: total weight of the mixture: 1 g; temperature: 80 °C; pO2: 1 barg; stirring speed: 1,000 r.p.m.; Key★: pure benzaldehyde;▴: 98% benzaldehyde and 2% benzyl alcohol; •: 90% benzaldehyde and 10% benzyl alcohol; ▪: 75% benzaldehyde and 25% benzyl alcohol. Data set for the same set of experiments for longer duration are presented inSupplementary Fig. 1. We reasoned that benzyl alcohol was probably acting to quench free radicals involved in autoxidation of benzaldehyde and that related molecules should act similarly (see Table 1 ). Replacing benzyl alcohol (hereafter labelled Ph-CH 2 OH) by an allylic alcohol, such as prenyl alcohol (3-methyl-2-buten-1-ol), was found to act in a similar way. Figure 1: Effect of benzyl alcohol on the aerobic oxidation of benzaldehyde. Reaction conditions: total weight of the mixture: 1 g; temperature: 80 °C; pO 2 : 1 barg; stirring speed: 1,000 r.p.m. ; Key ★ : pure benzaldehyde; ▴ : 98% benzaldehyde and 2% benzyl alcohol; •: 90% benzaldehyde and 10% benzyl alcohol; ▪: 75% benzaldehyde and 25% benzyl alcohol. Data set for the same set of experiments for longer duration are presented in Supplementary Fig. 1 . Full size image Table 1 Substrates that inhibit the autoxidation of benzaldehyde to benzoic acid*. Full size table Likewise, triphenylmethane, which was also readily convertible into the corresponding carbon-centred radical, was able to quench the autoxidation whereas toluene and methanol, possessing less activated hydrogen atoms, did not. 2-Phenyl-2-propanol, which is devoid of benzylic C–H groups, also did not inhibit benzoic acid formation. Most significantly, addition of phenyl-N- tert -butylnitrone (PBN), a well-known spin-trapping agent commonly used in EPR spectroscopy (see later), was very effective in suppressing autoxidation. Full details of the findings for all molecules investigated, and their structural motifs, are given in Table 1 . In all cases where suppression of the over-oxidation of the aldehyde is observed, the evidence points to inhibition by interception of free radicals involved in radical chain autoxidation by hydrogen atom transfer or, in the case of PBN, by addition to the C=N bond. The reactivity of the radicals so produced is then insufficient to sustain the autoxidation chain. We have confirmed that benzaldehyde readily undergoes autoxidation via a free radical chain mechanism. The reaction is known to be facilitated by Mn 3+ , Cu 2+ or Co 2+ salts, which presumably promote the initiation step [30] . Furthermore, certain additives inhibit benzaldehyde oxidation, suggesting that they interfere with the free radical processes. To investigate the free radicals involved in this mechanism in more detail, we employed the EPR spin trapping methodology using two nitrone-based traps: PBN and 5,5-dimethyl-1-pyrroline-N-oxide (DMPO), notwithstanding the known direct reaction of PBN with aldehydes [31] . Recently, Chechik and co-workers [20] have also demonstrated the utility of the spin trapping approach to characterize the radical intermediates involved in the Au nanoparticle-catalysed oxidation of aldehydes. EPR studies EPR spectra for anaerobic and aerobic benzaldehyde solutions containing the PBN-spin trap were recorded, both in the absence or presence of increasing benzyl alcohol concentrations. The resulting experimental and simulated spectra are given in Supplementary Fig. 2 . Under anaerobic conditions, two PBN-spin adducts (I and II) were detected, and in the presence of benzyl alcohol, the radical responsible for adduct I was selectively removed, leaving adduct II and weak signals of a new spin adduct V. By comparison, under aerobic conditions, two new PBN-spin adducts (III and IV) were detected, and once again in the presence of benzyl alcohol, one of these adducts (III) was selectively removed and replaced by traces of V. Traces of the fifth PBN-spin adduct (V), were detected in all solutions containing benzyl alcohol. On the basis of these EPR results, it appears that benzyl alcohol selectively removes one of the radicals normally present during autoxidation, thereby inhibiting the reaction. Importantly, addition of 2-phenyl-2-propanol to a benzaldehyde solution containing PBN, produced a strong signal attributed to spin adduct IV ( Supplementary Fig. 3 ). A complementary series of experiments were also conducted under identical conditions using DMPO ( Supplementary Fig. 4 ) and 2-methyl-2-nitrosopropane (MNP) ( Supplementary Fig. 5 ). For clarity, a detailed EPR discussion of the radical assignments (and mode of trapping as summarized in Supplementary Fig. 6 ) is given in the Supplementary Discussion . We interpret these experimental EPR observations in terms of the competitive reactions of radical intermediates involved in the radical chain oxidation of benzaldehyde. The reaction scheme that provides a coherent picture of the chain process occurring is illustrated in Fig. 2 . 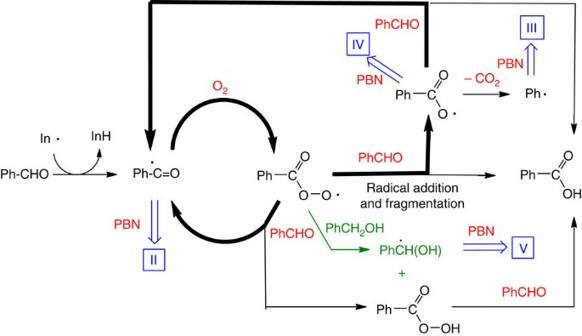Figure 2: Proposed reaction scheme for benzaldehyde autoxidation. Bold arrows indicate the main radical chain processes, while blue arrows represent the formation of the PBN-spin adducts II, III, IV and V. Key: In·: radical initiator. Figure 2: Proposed reaction scheme for benzaldehyde autoxidation. Bold arrows indicate the main radical chain processes, while blue arrows represent the formation of the PBN-spin adducts II, III, IV and V. Key: In · : radical initiator. Full size image The principal steps indicated in the main chain in Fig. 2 are: (i) initiation, resulting in the generation of carbon-centred benzoyl radicals, PhCO · ; (ii) capture of benzoyl radicals by molecular oxygen giving benzoylperoxy radicals, PhC(O)-OO · ; (iii) reaction of benzoylperoxy radicals with benzaldehyde to form perbenzoic acid, together with another benzoyl radical that then continues the chain. Perbenzoic acid is known to react with aldehydes in a non-radical Baeyer–Villiger-type oxidation, which in the present instance affords 2 moles of benzoic acid [32] . On this basis, it would appear that during the autoxidation of pure benzaldehyde, a number of radical species are generated, some of which are trapped since four distinct nitroxyl radicals were experimentally detected: two under anaerobic conditions (I and II) and two in the presence of oxygen (III and IV). Spin adduct I, observed only under anaerobic conditions, is an artefact not connected with the main autoxidation reaction and is believed to be a nitroxyl radical generated by nucleophile addition to PBN followed by oxidation [33] . On the other hand spin adduct II, also detected under anaerobic conditions, can be easily assigned to the benzoyl radical (PhCO · ) [34] , [35] . Under subsequent aerobic conditions, a competition for the benzoyl radicals arises between PBN and dioxygen; since adduct II is no longer detected under the aerobic conditions, it is evident that oxygen trapping dominates. Furthermore, a spin adduct assigned to a trapped benzoyl radical was also detected using DMPO ( Table 2 and Supplementary Fig. 4 ). Spin adducts III and IV can be assigned to the trapped phenyl (Ph · ) and benzoyloxy (PhC(O)-O · ) [35] , [36] radicals, respectively. According to Fig. 2 , oxygen addition to the benzoyl radical should produce the benzoylperoxy radical PhC(O)-OO · . However, while the PBN adducts of the benzoyloxy radical are well known [32] , [36] , [37] (see Table 2 ), the benzoylperoxy radical has never been reported. Alkylperoxy radical adducts with PBN are generally unstable at temperatures above 273 K, when they give rise to alkoxy adducts [38] , [39] , [40] . In the present experiments, conducted at 353 K, an analogous transformation would convert the benzoylperoxy adduct to the benzoyloxy adduct. Furthermore, a DMPO-spin adduct, which is consistent with the trapping of benzoyloxy radicals, was also observed ( Table 2 , Supplementary Fig. 4 ). Therefore, although we have no direct evidence for the formation or trapping of benzoylperoxy radicals by EPR, the circumstantial evidence for their formation is, we believe, overwhelming. Table 2 EPR hyperfine splittings for the PBN and DMPO adducts in benzaldehyde under aerobic and anaerobic conditions. Full size table As discussed above, the PhCO-O-PBN adduct may originate, at least in part, by the thermal decomposition of the PhCO-OO-PBN adduct under the adopted experimental conditions. An alternative possibility for formation of benzoyloxy radicals is via reaction of benzoylperoxy radicals with benzaldehyde ( Fig. 2 ). In competition with H-abstraction from the solvent, the benzoylperoxy radicals may add to the carbonyl function yielding an adduct that rearranges and fragments into a molecule of benzoic acid and a benzoyloxy radical (see Fig. 3 ). In the absence of inhibitors and spin traps, the benzoyloxy radicals can abstract hydrogen from benzaldehyde to complete a supplementary autoxidation cycle. This H-abstraction would have to compete successfully with the loss of carbon dioxide (rate constant of the order of 10 6 s −1 ) leading to the formation of a phenyl radical (Ph · ). In fact, the PBN-spin adduct III ( Table 2 ) can be easily assigned to a trapped phenyl radical, generated from benzoyloxy radicals by loss of CO 2 on a timescale of microseconds (see Fig. 2 ). 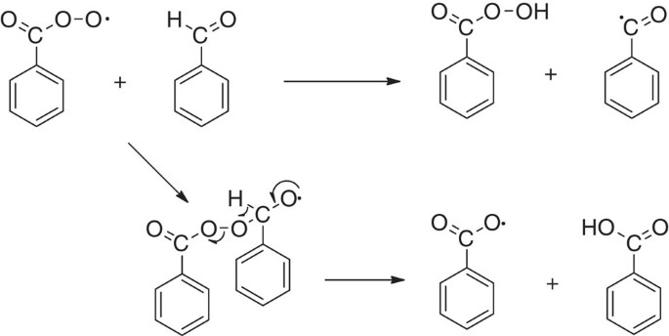Figure 3: Proposed competing reactions of benzoylperoxy radicals with benzaldehyde.  Figure 3: Proposed competing reactions of benzoylperoxy radicals with benzaldehyde. Full size image We believe that benzyl alcohol and other inhibitors intercept intermediate radicals in competition with radical reactions that form an integral part of the autoxidation cycle. In the absence of oxygen, benzoyl radicals are formed and benzyl alcohol merely reduces the intensity of the EPR signal attributed to the benzoyl-PBN adduct ( Supplementary Fig. 2 ). This arises by H-transfer from the benzylic C–H groups, reforming benzaldehyde and generating rather unreactive α-hydroxybenzyl radicals, PhCH(OH) · , that can be oxidized to benzaldehyde or disproportionate to benzaldehyde plus benzyl alcohol. The hydroxybenzyl radical was indeed easily identified using PBN added to pure benzyl alcohol ( Table 2 ); PBN-spin adducts of this trapped hydroxybenzyl radical were also detected in benzaldehyde solutions containing benzyl alcohol, both in anaerobic and aerobic conditions ( Supplementary Fig. 2 ). On the basis of the simulations of the EPR spectra, small contributions (~20%) from this PhCH(OH) · radical adduct were detected in the benzaldehyde solutions containing 2 and 10% benzyl alcohol ( Supplementary Fig. 2b,c ); these spectra were dominated by major contributions (~80%) from the benzoyl radical adducts. It is important to note that the overall abundance of the α-hydroxybenzyl radical trapped by PBN (adduct V) is much larger in the benzaldehyde solutions ( Supplementary Fig. 2b,c ) compared with the pure benzyl alcohol ( Supplementary Fig. 2d ). The effect of oxygen is then evidently to transform benzoyl radicals rapidly into O-centred radicals ( Supplementary Fig. 2e–h ). In the absence of benzyl alcohol ( Supplementary Fig. 2e ) two different adducts were detected, that is, adduct III (phenyl) with ~25% relative abundance and adduct IV (benzoyloxy) with ~75% relative abundance. However, in the presence of benzyl alcohol, only adducts IV and V were observed ( Supplementary Fig. 2f,g ), that is, adduct IV (benzoyloxy) with ~45% abundance and adduct V (α-hydroxybenzyl) with ~45% abundance along with a smaller residual (≤10%) contribution from adduct III. We have proposed ( Fig. 2 ) that the two O-centred radicals are produced sequentially but only the spin adduct of PhCO-O · is actually detected. This might imply that PBN is not an efficient trap for the precursor benzoylperoxy radicals in competition with their reaction with the benzaldehyde solvent. This is not unreasonable since it is known [41] that the rate constants for PBN trapping of peroxy radicals under conditions similar to those used in this investigation are rather low, and for the benzoyloxy radical is several orders of magnitude greater (4 × 10 5 M −1 s −1 at 40 °C in benzene solution) [42] . In addition, the PhCO-O-PBN adducts could be derived by decomposition of PhCO-OO-PBN by analogy with the ROO-PBN→RO-PBN transformation, as discussed earlier. Upon addition of benzyl alcohol, H-transfer to benzoylperoxy and benzoyloxy radicals is enhanced, reducing the proportion of the latter losing CO 2 to yield phenyl radicals as trapped by PBN (adduct III) to below the detection limit. Nevertheless, some benzoyloxy radicals are trapped by PBN as adduct IV. We consider that our work provides new insight into the longstanding mystery surrounding inhibition of benzaldehyde oxidation. In particular, we have shown that benzyl alcohol is a very effective inhibitor by virtue of its ability to act as a hydrogen atom donor, thereby explaining why oxidation of the alcohol under a variety of conditions can lead to formation of benzaldehyde in high yield, with little further oxidation to benzoic acid. To conclude, in the aerobic oxidation of benzyl alcohol to benzaldehyde, in spite of its facile oxidizable nature, benzaldehyde is obtained mostly in high yield (~99%), even in the presence of highly oxidizing environments. This has long been an unsolved mystery. Here, with the aid of EPR spin trapping experiments, we show that benzyl alcohol (even as little as 2 wt%) quenches the oxidation of benzaldehyde to benzoic acid principally by intercepting the acylperoxy radicals, which are responsible for the oxidation of benzaldehyde to benzoic acid. Testing of several alcohols, in place of benzyl alcohol, reveals that alcohols with at least one benzylic or allylic α-H quenches the oxidation of benzaldehyde to benzoic acid. Our preliminary experiments, shown in Fig. 4 , reveal surprisingly that 1-octanol has an analogous inhibiting effect on the autoxidation of octanal. Further quantitative investigation is necessary before it can be claimed that this behaviour is generic. The inhibitory effect of benzyl alcohol on benzaldehyde autoxidation is associated with the low bond dissociation energy of C–H bonds in the α-position relative to the hydroxyl group, enhanced since the α-Hs are also benzylic. In wholly aliphatic systems a hydroxyl group certainly lowers the bond strength of an α-C–H bond substantially, compared with the parent hydrocarbon but a C–H bond adjacent to a –CHO group is even weaker. 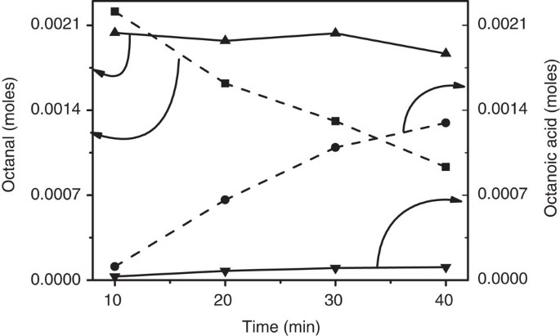Figure 4: Inhibition of the aerobic auto oxidation of octanal by 1-octanol. Time online data for the oxidation of 100% octanal (dashed line) and 90 wt % octanal+10 wt% 1-octanol (solid line) are presented here. Key: ▪: moles of octanal for 100% octanal reaction; •: moles of octanoic acid for 100% octanal reaction;▴: moles of octanal for 90 wt% octanal+10 wt% octanol reaction;▾: moles of octanoic acid for 90 wt% octanal+10 wt% octanol reaction: reaction conditions: 2 g of substrate; T: 353 K; pO2: 1 barg; stirring speed; 1,000 r.p.m. Figure 4: Inhibition of the aerobic auto oxidation of octanal by 1-octanol. Time online data for the oxidation of 100% octanal (dashed line) and 90 wt % octanal+10 wt% 1-octanol (solid line) are presented here. Key: ▪: moles of octanal for 100% octanal reaction; •: moles of octanoic acid for 100% octanal reaction; ▴ : moles of octanal for 90 wt% octanal+10 wt% octanol reaction; ▾ : moles of octanoic acid for 90 wt% octanal+10 wt% octanol reaction: reaction conditions: 2 g of substrate; T: 353 K; pO 2 : 1 barg; stirring speed; 1,000 r.p.m. Full size image Materials Benzaldehyde, benzoic acid, benzyl alcohol, methanol, toluene, triphenylmethane, 3-methyl-2-buten-1-ol, 2-phenyl-2-propanol, PBN, DMPO and MNP were purchased from Sigma Aldrich and used without any further treatment. Oxidation reactions and analysis All the oxidation reactions were carried out in a 50 ml moderate pressure, glass reactor stirred using a magnetic bar. In a typical reaction, the requisite amount of additive and substrate was charged into the reactor, which was then purged with the O 2 three times before closing and the pressure was maintained at 1 bar (relative pressure). The reactor with the reaction mixture was kept in a preheated heating block, which was maintained at the reaction temperature. The reaction mixture was then stirred using a magnetic bar inside the reactor at 1,000 r.p.m. After a specific time, the stirring was stopped and the reactor was cooled in an ice bath immediately. The slurry containing crystalline material was mixed with 1 ml of acetone to obtain homogeneous liquid. A 0.5 ml of this aliquot was added to 0.5 ml of mesitylene (external standard for GC analysis). Separate reactions were carried out for one particular point in the kinetic plot. The kinetic plot for one reaction was obtained by five different reactions that were stopped at different time intervals. For the analysis of the products, GC–MS (Waters, GCT Premier) and GC (a Varian star 3800 cx with a 30 m CP-Wax 52 CB column) were employed. The products were identified by comparison with known standards. For the quantification of the amounts of reactants consumed and products generated, an external calibration method was used. EPR experiments X-band continuous wave EPR spectra were recorded at room temperature in deoxygenated and oxygenated benzaldehyde solutions using a Bruker EMX spectrometer. The typical instrument parameters were; centre field 3345 G, sweep width 50 G, sweep time 55 s, time constant 10 ms, MW power 5 mW, modulation 100 kHz and modulation amplitude 1 G. Spectral simulations were obtained using the commercially available Bruker SIMFONIA software programme. For spectral measurements, different concentrations of the PBN and DMPO solutions were used, ranging from 2–200 mg of spin trap. Typically the larger concentrations were used to trap all observable adducts. How to cite this article: Sankar, M. et al. The benzaldehyde oxidation paradox explained by the interception of peroxy radical by benzyl alcohol. Nat. Commun. 5:3332 doi: 10.1038/ncomms4332 (2014).